Induction and reversal of myotonic dystrophy type 1 pre-mRNA splicing defects by small molecules The ability to control pre-mRNA splicing with small molecules could facilitate the development of therapeutics or cell-based circuits that control gene function. Myotonic dystrophy type 1 is caused by the dysregulation of alternative pre-mRNA splicing due to sequestration of muscleblind-like 1 protein (MBNL1) by expanded, non-coding r(CUG) repeats (r(CUG) exp ). Here we report two small molecules that induce or ameliorate alternative splicing dysregulation. A thiophene-containing small molecule ( 1 ) inhibits the interaction of MBNL1 with its natural pre-mRNA substrates. Compound ( 2 ), a substituted naphthyridine, binds r(CUG) exp and displaces MBNL1. Structural models show that 1 binds MBNL1 in the Zn-finger domain and that 2 interacts with UU loops in r(CUG) exp . This study provides a structural framework for small molecules that target MBNL1 by mimicking r(CUG) exp and shows that targeting MBNL1 causes dysregulation of alternative splicing, suggesting that MBNL1 is thus not a suitable therapeutic target for the treatment of myotonic dystrophy type 1. Pre-mRNA splicing defects cause a wide variety of diseases including β-thalassaemia, inherited breast cancer, fragile X-associated tremor ataxia syndrome and myotonic dystrophy types 1 and 2 (DM1 and DM2, respectively) [1] , [2] , [3] , [4] , [5] , [6] . In the former two cases, pre-mRNA splicing defects are caused by single-nucleotide polymorphisms within intronic regions of their mRNAs, yielding cryptic alternative splice sites. In the latter three cases, pre-mRNA splicing defects are caused by sequestration of proteins that regulate alternative pre-mRNA splicing [5] , [7] . DM1 is caused by sequestration of muscleblind-like 1 protein (MBNL1) by expanded r(CUG) repeats (r(CUG) exp ) present in the 3′-untranslated region (UTR) of the dystrophia myotonica protein kinase ( DMPK ) mRNA [8] . r(CUG) exp folds into an extended hairpin that displays multiple copies of a 5′C U G/3′G U C motif, which are high-affinity-binding sites for MBNL1. Studies in patient-derived cell lines and in mouse models have shown that pre-mRNA splicing events are dysregulated in DM1, including alternative splicing of the insulin receptor (IR) [9] , cardiac troponin T (cTNT) [10] and the muscle-specific chloride ion channel ( CLCN1 ) [11] , [12] . These defects explain symptoms suffered by DM1 patients such as insulin insensitivity (IR splicing), myotonia ( CLCN1 splicing) and cardiac defects (cTNT splicing). Moreover, translational defects of the DMPK mRNA and the presence of nuclear foci are observed in DM patients [13] , [14] . Both defects are due to the binding of r(CUG) exp to various proteins, leading to poor nucleocytoplasmic transport [13] , [15] . To identify small molecules that disrupt the r(CUG) exp –MBNL1 complex, we previously developed an assay amendable for quantitative high-throughput screening [16] . The small molecules that comprise the Molecular Libraries Small Molecule Repository (>300,000 members) were screened, and the results have been published online at PubChem ( http://pubchem.ncbi.nlm.nih.gov/assay/assay.cgi?aid=2675&loc=ea_ras ) and in Chen et al . [16] The high-throughput screen identifies compounds that inhibit the r(CUG)-MBNL1 interaction by binding the RNA or the protein. Thus, a small molecule that binds r(CUG) exp and displaces MBNL1 could theoretically improve DM1-associated pre-mRNA splicing defects ( Fig. 1a ). However, small molecules that bind MBNL1 and disrupt the r(CUG) exp –MBNL1 interaction may inactivate the protein and induce DM1-like pre-mRNA splicing defects ( Fig. 1a ). Importantly, the screen could yield chemotypes that reverse DM1-associated pre-mRNA splicing defects as a first step towards the development of therapeutics for this devastating disease. 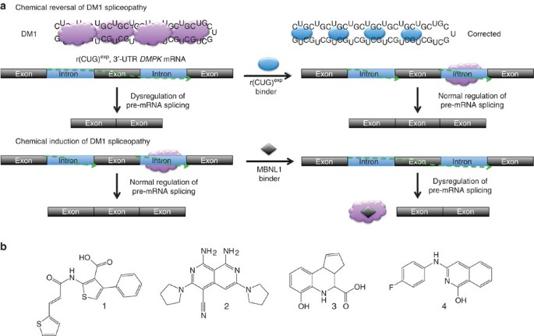Figure 1: Identification of small molecules that inhibit the formation of the r(CUG)12–MBNL1 complex. (atop) The biochemical outcome of a small molecule that targets r(CUG)expwould be the improvement of DM1-associated pre-mRNA splicing defects. (abottom) The biochemical outcome of a small molecule that targets MBNL1 would be the induction of DM1-associated pre-mRNA splicing defects. (b) The small molecules that inhibit formation of the r(CUG)12–MBNL1 complex as identified by screening of the NIH’s MLPCN library. Figure 1: Identification of small molecules that inhibit the formation of the r(CUG) 12 –MBNL1 complex. ( a top) The biochemical outcome of a small molecule that targets r(CUG) exp would be the improvement of DM1-associated pre-mRNA splicing defects. ( a bottom) The biochemical outcome of a small molecule that targets MBNL1 would be the induction of DM1-associated pre-mRNA splicing defects. ( b ) The small molecules that inhibit formation of the r(CUG) 12 –MBNL1 complex as identified by screening of the NIH’s MLPCN library. Full size image Herein, we describe the results from our investigation of two hits from our quantitative high-throughput screening: one that reverses DM1 pre-mRNA spliceopathy and another that induces DM1-like pre-mRNA spliceopathy. These compounds can serve as useful tools to study the effect of DM1 splicing on disease and to understand how to control pre-mRNA splicing or translation with cell-permeable small molecules. High-throughput screening for lead compounds against DM1 Previously, our team reported a screen for inhibitors of the toxic RNA–protein interaction that causes myotonic dystrophy type 1 (DM1) (ref. 16 ). The screen was designed to identify ligands that inhibit formation of a r(CUG)–MBNL1 complex that causes DM1. The assay utilizes biotinylated r(CUG) 12 and MBNL1-His 6 . After formation of the RNA–protein complex, a ligand of interest is added followed by the addition of fluorescently labelled streptavidin (recognizes biotinylated r(CUG) 12 ) and a fluorescently labelled anti-His 6 antibody (recognizes MBNL1). When the r(CUG) 12 –MBNL1 complex forms, the two fluorophores are within close enough proximity to form a fluorescence resonance energy transfer (FRET) pair, and time resolved (TR)-FRET can be measured. If, however, a small molecule inhibits r(CUG) 12 –MBNL1 complex formation, no TR-FRET would be observed. Four compounds identified from the NIH Chemical Genomics Center (NCGC) screen were further investigated: (E)-4-phenyl-2-(3-(thiophen-2-yl)acrylamido)thiophene-3-carboxylic acid ( 1 ), 1,8-diamino-3,6-di(pyrrolidin-1-yl)-2,7-naphthyridine-4-carbonitrile ( 2 ), 6-hydroxy-3a,4,5,9b-tetrahydro-3H-cyclopenta[c]quinoline-4-carboxylic acid ( 3 ), and 3-((4-fluorophenyl)amino)isoquinolin-1-ol ( 4 ) ( Fig. 1b ). These compounds inhibit formation of the r(CUG) 12 –MBNL1 complex with IC 50 ’s that range from 2–242 μM when the ligand and RNA are incubated first followed by addition of MBNL1. Compounds 2 and 3 are the most and least potent, respectively ( Table 1 ). Table 1 Potencies and selectivities of compounds 1 – 4 *. Full size table Improvement of DM1-associated translational defects As an initial test for bioactivity, a previously described cellular model system that mimics the DMPK translational defects observed in DM1 was used ( Fig. 2a , ref. 17 ). In this model, firefly luciferase mRNA containing 800 r(CUG) repeats (r(CUG) 800 ) in the 3′-UTR is stably expressed in C2C12 cells. Formation of the r(CUG) 800 –MBNL1 complex retains the firefly luciferase mRNA in the nucleus, disallowing nucleocytoplasmic transport. If a small molecule enters the nucleus and displaces MBNL1 from r(CUG) 800 , then the luciferase mRNA may be translocated to the cytoplasm and translated, resulting in increased luciferase activity. An increase in luciferase activity should be observed if compounds bind to r(CUG) exp or MBNL1, as both inhibit the formation of the r(CUG) 800 –MBNL1 complex. 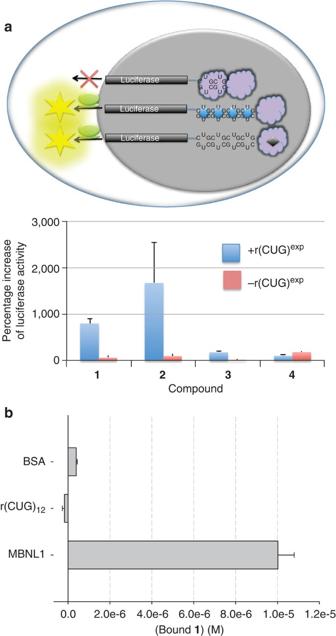Figure 2: Compounds1–4improve translational defects caused by r(CUG)exp. Improvement of translational could occur if a compound binds to r(CUG)exp(compound2) or MBNL1 (compound1), as both modes of action disrupt the r(CUG)exp–MBNL1 complex and could allow for more efficient nucleocytoplasmic export. (a, top) A schematic of the luciferase reporter system that models the DM1 translational defect. The presence of r(CUG)expin the 3′-UTR of firefly luciferase reduces nucleocytoplasmic transport and thereby suppresses luciferase expression. However, if a small molecule binds r(CUG)expand displaces proteins, nucleocytoplasmic transport is improved and luciferase activity increases. Likewise, if a small molecule binds proteins and displaces them from r(CUG)exp, nucleocytoplasmic transport is also improved and luciferase activity increases. (a, bottom) Effects on luciferase activity when cells are dosed with 20 μM compound of interest. ‘+r(CUG)exp’ indicates that the cell line expresses luciferase with r(CUG)expin the 3′-UTR, ‘-r(CUG)exp’ indicates that the cell line expresses luciferase without r(CUG)exp. Results are expressed as the percentage increase of luciferase activity relative to untreated cells, where a value of ‘0’ denotes no change in activity. Experiments were completed in triplicate. Values shown in the plot are the averages of those experiments, and the errors reported are the s.d. values. (b) Competition dialysis data for binding of1to BSA, MBNL1 and r(CUG)12. The data clearly show that the preferred target is MBNL1 as there is no measureable binding to r(CUG)12or to BSA. Experiments were completed in duplicate. The values reported are the averages of those experiments, and the errors reported are the s.d. values. Figure 2: Compounds 1 – 4 improve translational defects caused by r(CUG) exp . Improvement of translational could occur if a compound binds to r(CUG) exp (compound 2 ) or MBNL1 (compound 1 ), as both modes of action disrupt the r(CUG) exp –MBNL1 complex and could allow for more efficient nucleocytoplasmic export. ( a , top) A schematic of the luciferase reporter system that models the DM1 translational defect. The presence of r(CUG) exp in the 3′-UTR of firefly luciferase reduces nucleocytoplasmic transport and thereby suppresses luciferase expression. However, if a small molecule binds r(CUG) exp and displaces proteins, nucleocytoplasmic transport is improved and luciferase activity increases. Likewise, if a small molecule binds proteins and displaces them from r(CUG) exp , nucleocytoplasmic transport is also improved and luciferase activity increases. ( a , bottom) Effects on luciferase activity when cells are dosed with 20 μM compound of interest. ‘+r(CUG) exp ’ indicates that the cell line expresses luciferase with r(CUG) exp in the 3′-UTR, ‘-r(CUG) exp ’ indicates that the cell line expresses luciferase without r(CUG) exp . Results are expressed as the percentage increase of luciferase activity relative to untreated cells, where a value of ‘0’ denotes no change in activity. Experiments were completed in triplicate. Values shown in the plot are the averages of those experiments, and the errors reported are the s.d. values. ( b ) Competition dialysis data for binding of 1 to BSA, MBNL1 and r(CUG) 12 . The data clearly show that the preferred target is MBNL1 as there is no measureable binding to r(CUG) 12 or to BSA. Experiments were completed in duplicate. The values reported are the averages of those experiments, and the errors reported are the s.d. values. Full size image All four compounds shown in Fig. 1b were tested in this system at 20 μM ( Fig. 2a ). Compounds 1 and 2 stimulated luciferase production most effectively, with increases in luciferase activity of ~700% and ~1,600%, respectively. (Please note that no change in luciferase activity is equal to 0%.) Compounds 3 and 4 also increase luciferase activity but to a lesser extent (ca. 125%). Control experiments were completed using an analogous cellular model system that stably expresses firefly luciferase mRNA lacking r(CUG) exp . A slight increase in luciferase activity was observed for compounds 1 , 2 and 3 , although the increase is small compared to the increase observed in the presence of r(CUG) exp . In the case of compound 4 , however, we observed similar increases in luciferase activity in cell lines with and without r(CUG) exp , indicating a nonspecific effect. Therefore, 4 was no longer pursued as a lead compound. Owing to the enhanced biological activity of 1 and 2 , these two compounds were further investigated. Affinity and selectivity of 1 and 2 for r(CUG) exp and MBNL1 The binding of 1 and 2 to a mimic r(CUG) exp , r(CUG) 12 , and MBNL1 were determined by competition dialysis [18] and fluorescence anisotropy, respectively. Compound 2 nonspecifically adheres to dialysis membranes, and thus is incompatible with competition dialysis. Competition dialysis shows that 1 binds specifically to MBNL1 over both r(CUG) 12 and a protein control, bovine serum albumin (BSA) ( Fig. 2b ). Almost no detectable partitioning of 1 was observed into dialysis tubes that contained BSA or r(CUG) 12 . In contrast, a large amount of partitioning was observed in tubes that contained MBNL1, affording a K d of 470±20 nM. These data suggest that 1 inhibits r(CUG) exp –MBNL1 complex formation by binding to MBNL1 ( Fig. 1a ). Fluorescence anisotropy measurements with 2 show that it binds specifically to r(CUG) 12 with a K d of 125 nM and a stoichiometry of ~6 small molecules per RNA ( Table 2 ). No change in anisotropy was observed when up to two times the concentration of MBNL1 (650 nM) and ~35 times the concentration of BSA (12.5 μM) were added to 2 (325 nM), indicating weak protein binding. The affinity of 2 for another repeating RNA, r(CAG) 12 ( Supplementary Fig. S1 ), and a fully paired RNA ( AU , Supplementary Fig. S1 ) were also determined. Compound 2 binds r(CAG) 12 with a dissociation constant of 1,400 nM and a 1:1 stoichiometry while no binding was observed to the AU RNA ( K d >> 25,000 nM) ( Table 2 ). Table 2 Affinity of 2 for various biomolecules. Full size table The binding of 2 to an RNA containing a single 1 × 1 nucleotide UU internal loop ( 1 × 1 UU , Supplementary Fig. S1 ) was also measured. The compound binds 1 × 1 UU with a 1:1 stoichiometry and a K d of 500 nM. There is an ~4-fold difference in affinity of 2 for r(CUG) 12 and 1 × 1 UU . These data suggest that the ligand binds with positive cooperativity to longer RNAs. Such properties are favourable for selectively recognizing r(CUG) exp in vivo [19] as many other genomic RNA targets contain single 1 × 1 nucleotide UU internal loop, notably the A-site in human ribosomes. Selectivity of 1 and 2 for inhibiting RNA–MBNL1 complexes As 1 binds to MBNL1, its potency for disrupting RNA–MBNL1 interactions should be independent of the RNA’s sequence. In contrast, 2 (binds specifically to r(CUG) exp ) should more potently inhibit r(CUG) 12 –MBNL1 complex formation as compared with complexes formed with other RNAs that bind MBNL1 (r(CAG) 12 , r(CCUG) 12 and r(CGG) 12 , for example refs 20 , 21 . (r(CAG) exp –MBNL1 and r(CCUG) exp –MBNL1 complexes cause pre-mRNA splicing defects in Huntington disease patient-derived cell lines and in a myotonic dystrophy type 2 cellular model, respectively [2] , [6] , [15] , [22] .) Therefore, we studied the potencies of compounds 1 and 2 for preventing RNA–MBNL1 complex formation ( Table 1 ). In these experiments, 1 was pre-incubated with MBNL1, followed by addition of RNA while 2 was pre-incubated with the RNA of interest followed by addition of MBNL1. As expected, our results indicate that compound 1 is a general inhibitor of RNA–MBNL1 complexes with an average IC 50 of 62±10 μM ( Table 1 ). In contrast, the IC 50 ’s for 2 vary from 2 μM (r(CUG) 12 ) to 45 μM (r(CGG) 12 ). Compound 2 is at least 10-fold more potent for inhibiting the r(CUG) 12 –MBNL1 interaction than for inhibiting r(CAG) 12 -, r(CCUG) 12 - and r(CGG) 12 –MBNL1 interactions. These data are in good agreement with the results of the binding measurements summarized in Table 2 and Fig. 2b and further support the hypothesis that the potencies of 1 and 2 are derived from binding MBNL1 and r(CUG) exp , respectively. The contrasting modes of in vitro inhibition and binding data support the results observed in the luciferase assay. The luciferase model system cannot discriminate between compounds that disrupt r(CUG) exp –protein complexes by binding r(CUG) exp from those that disrupt the complexes by binding to proteins. If a small molecule binds to either protein or RNA, then the complex will be disrupted, allowing the mRNA to be translocated to the cytoplasm and translated. Our previously described competition dialysis, anisotropy and potency data suggest that compounds 1 and 2 could have very different effects on pre-mRNA splicing. Compound 1 , which binds MBNL1, could prevent MBNL1 from binding to its natural pre-mRNA substrates, inducing DM1-like splicing dysregulation in non-DM1 cells (that is, like that observed when MBNL1 is sequestered by r(CUG) exp ) ( Fig. 1a ). Compound 2 , which binds r(CUG) exp , may displace MBNL1, freeing it to regulate pre-mRNA splicing as though r(CUG) exp had been removed ( Fig. 1a ). Compound 1 induces splicing defects MBNL1 regulates the alternative splicing of many pre-mRNAs [7] , [9] , [10] , [11] , [12] , [23] , [24] . Numerous splicing defects are observed in DM1 patients including the IR and the cTNT pre-mRNAs [9] , [10] , [23] , [24] . It has been shown that co-transfection of HeLa cells with a DM1 mini-gene that expresses 960 interrupted r(CUG) repeats causes dysregulation of mini-genes regulated by MBNL1; in particular splicing defects in the IR and cTNT pre-mRNAs have been observed by reverse transcription PCR (RT–PCR) [10] , [20] , [25] , [26] . The percentage of exon 11 included in the IR mini-gene transcripts decreases from ≈97% in the absence of r(CUG) exp to ≈75% in the presence of r(CUG) exp ( Fig. 3 ). Regarding the alternative splicing of the cTNT pre-mRNA, the percentage of exon 5 inclusion increases from ≈75% in the absence of r(CUG) exp to ≈90% in the presence of r(CUG) exp ( Fig. 3 ). 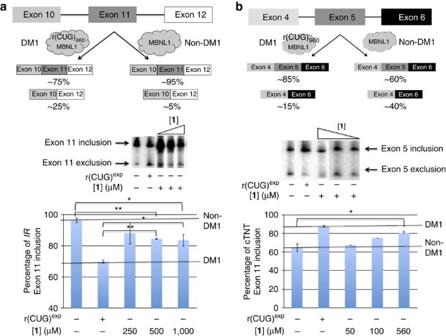Figure 3: Compound1induces DM1-like splicing defects in HeLa cells. HeLa cells were co-transfected with the mini-gene of interest and a plasmid that expresses r(CUG)expor an empty vector. Varying concentrations of1were added in growth medium post transfection, and total RNA was harvested 16–20 h later. The percentage of each splicing isoform was determined by RT–PCR using a radioactively labelled forward PCR primer. (a, top) Schematic of the pre-mRNA splicing isoforms observed for the IR mini-gene. (a, middle) representative gel image of IR alternative splicing in the presence of varying concentrations of1. (a, bottom) Quantification of exon inclusion for IR alternative splicing in the presence or absence of r(CUG)expand1(n≥3). Error bars are the s.d. values in the measurements. (b, top) Schematic of the pre-mRNA splicing isoforms observed for the cTNT mini-gene. (b, middle) representative gel image of cTNT alternative splicing in the presence of varying concentrations of1. (b, bottom) Quantification of exon inclusion for cTNT alternative splicing in the presence or absence of r(CUG)expand1(n≥3). Error bars are the s.d. values in the measurements. ‘*’ indicatesP≤0.05 and ‘**’ indicatesP≤0.01 as determined by a two-tailed Student’st-test. Figure 3: Compound 1 induces DM1-like splicing defects in HeLa cells. HeLa cells were co-transfected with the mini-gene of interest and a plasmid that expresses r(CUG) exp or an empty vector. Varying concentrations of 1 were added in growth medium post transfection, and total RNA was harvested 16–20 h later. The percentage of each splicing isoform was determined by RT–PCR using a radioactively labelled forward PCR primer. ( a , top) Schematic of the pre-mRNA splicing isoforms observed for the IR mini-gene. ( a , middle) representative gel image of IR alternative splicing in the presence of varying concentrations of 1 . ( a , bottom) Quantification of exon inclusion for IR alternative splicing in the presence or absence of r(CUG) exp and 1 (n≥3). Error bars are the s.d. values in the measurements. ( b , top) Schematic of the pre-mRNA splicing isoforms observed for the cTNT mini-gene. ( b , middle) representative gel image of cTNT alternative splicing in the presence of varying concentrations of 1 . ( b , bottom) Quantification of exon inclusion for cTNT alternative splicing in the presence or absence of r(CUG) exp and 1 ( n ≥3). Error bars are the s.d. values in the measurements. ‘*’ indicates P ≤0.05 and ‘**’ indicates P ≤0.01 as determined by a two-tailed Student’s t -test. Full size image Treatment of HeLa cells that do not express r(CUG) exp with compound 1 causes a shift in the alternative splicing patterns of the IR and cTNT mini-genes towards a DM1-like phenotype ( Fig. 3 ). Dysregulation of IR pre-mRNA splicing is observed when cells are treated with 500 and 1,000 μM of 1 . Likewise, alternative splicing of the cTNT mini-gene is shifted towards DM-like phenotype when cells are dosed with compound 1 , and a dose–response is observed from 50 to 560 μM. Statistically significant changes in cTNT alternative splicing are only observed at 560 μM when compared with cells that do not express r(CUG) exp . In order to determine if compound 1 generally affects the regulation of alternative splicing, additional experiments were completed with three mini-genes, the alternative splicing of which are not controlled by MBNL1 ( Supplementary Fig. S2 a-c) [5] , [26] , [27] , [28] (refs 5 , 26 , 27 , 28 ). These include pleckstrin homology domain containing, family H member 2 ( PLEKHH2 ) ref. 26 , survival of motor neuron 2 ( SMN2 ) (ref. 28 ) and B-cell lymphoma x (Bcl-x ) [27] . The alternative splicing of SMN2 and Bcl-x is regulated by the pre-mRNA splicing regulatory protein Sam68 (ref. 5 ). Sam68 is sequestered by r(CGG) exp in Fragile X-associated tremor ataxia syndrome, causing dysregulation of SMN2 and Bcl-x alternative splicing [5] . HeLa cells were co-transfected with the splicing reporter of interest and a DM1 mini-gene or a mini-gene that expresses only five r(CUG) repeats. Exposure of transfected cells to 500 μM of 1 had no effect on alternative splicing of PLEKHH2 or Bcl-x ( Supplementary Fig. S2 a,c). A modest change in SMN2 alternative splicing was observed when cells were treated with 1 but this effect was independent of r(CUG) exp ( Supplementary Fig. S2 B). Taken together, 1 primarily affects pre-mRNA splicing of genes controlled by MBNL1 but not those controlled by other proteins. Next, we tested the effect of 1 on normal and DM1-affected human fibroblasts. Normal human fibroblasts were treated with 1 for 48 h, and its effect on the splicing of several MBNL1-dependent exons were determined including MBNL1 , muscleblind-like 2 ( MBNL2 ), nuclear receptor co-repressor 2 ( NCOR2 ), nuclear factor I/X (CCAAT-binding transcription factor) ( NFIX ), and calcium/calmodulin-dependent protein kinase II gamma ( CAMK2G ). Splicing abnormalities (towards the DM-like phenotype) were observed when cells were treated with 250 or 500 μM of 1 for all five MBNL1-dependent exons ( Fig. 4a ). The strongest effects were observed for MBNL1 and MBNL2 exons, in which splicing dysregulation is the same as in DM1 affected fibroblasts. The DM1-like splicing shift in NCOR2, NFIX and CAMK2G was also evident upon 500 μM 1 , although more subtle than in the case of MBNL s ( Fig. 4a ). 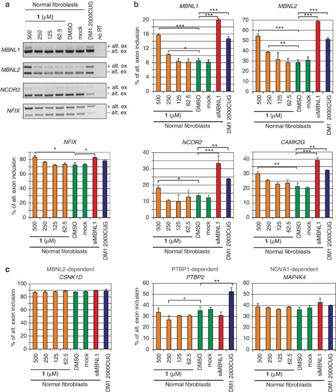Figure 4: Compound1induces an MBNL1-dependent DM1-like splicing shift in normal human fibroblasts. (a) Representative RT–PCR assays showing splicing changes in MBNL1-dependent exons in normal fibroblasts treated with increasing amounts of1(n=2). The DM1-like splicing shift is depicted as alternative exon inclusion (+alt. ex.), while the normal splicing isoform is depicted as alternative exon exclusion (-alt. ex). As a control, untreated and DMSO-treated (DMSO) normal fibroblasts (n=5) and DM1 fibroblasts expressing 2,000 CUG repeats (DM1 2000 CUG) (n=4) were used. No RT lane refers to RT–PCR control without reverse transcriptase. (b,c) Quantification of alternative splicing shift towards the DM1-like phenotype (% of alternative exon inclusion) in normal fibroblasts treated with increasing concentrations of1(orange bars;n=2), untreated and DMSO-treated normal fibroblasts (green bars;n=5), siMBNL1-treated normal fibroblasts (red bars;n=2) and DM1-affected human fibroblasts expressing 2,000 r(CUG) repeats (blue bars;n=2). Splicing of MBNL1-dependent exons is shown inbwhile splicing of MBNL1-independent exons is shown inc. Each sample was subjected to RT–PCR twice. The errors reported are the s.d. values derived from analysis of all samples. ‘*’ indicatesP≤0.05; ‘**’ indicatesP≤0.01; and ‘***’ indicatesP≤0.001 as determined by a two-tailed Student’st-test. Figure 4: Compound 1 induces an MBNL1-dependent DM1-like splicing shift in normal human fibroblasts. ( a ) Representative RT–PCR assays showing splicing changes in MBNL1-dependent exons in normal fibroblasts treated with increasing amounts of 1 ( n =2). The DM1-like splicing shift is depicted as alternative exon inclusion (+alt. ex. ), while the normal splicing isoform is depicted as alternative exon exclusion (-alt. ex). As a control, untreated and DMSO-treated (DMSO) normal fibroblasts ( n =5) and DM1 fibroblasts expressing 2,000 CUG repeats (DM1 2000 CUG) ( n =4) were used. No RT lane refers to RT–PCR control without reverse transcriptase. ( b , c ) Quantification of alternative splicing shift towards the DM1-like phenotype (% of alternative exon inclusion) in normal fibroblasts treated with increasing concentrations of 1 (orange bars; n =2), untreated and DMSO-treated normal fibroblasts (green bars; n =5), siMBNL1-treated normal fibroblasts (red bars; n =2) and DM1-affected human fibroblasts expressing 2,000 r(CUG) repeats (blue bars; n =2). Splicing of MBNL1-dependent exons is shown in b while splicing of MBNL1-independent exons is shown in c . Each sample was subjected to RT–PCR twice. The errors reported are the s.d. values derived from analysis of all samples. ‘*’ indicates P ≤0.05; ‘**’ indicates P ≤0.01; and ‘***’ indicates P ≤0.001 as determined by a two-tailed Student’s t -test. Full size image Notably, efficient short interfering RNA (siRNA) knockdown of MBNL1 (by ~70% relative to untreated controls) in normal fibroblasts triggered only slightly more pronounced DM1-like splicing shift in MBNL1-dependent exons than treatment with 1 or than DM1 affected fibroblasts ( Fig. 4b , Supplementary Fig. S3A ). This suggests that 500 μM of 1 is not a saturating concentration required to induce a maximum possible effect on the splicing activity of MBNL1. To explore whether compound 1 -induced DM-like splicing alterations can be further exacerbated, we next knocked-down MBNL1 in normal human fibroblasts using siRNA and then, 24 h post siMBNL1 transfection, treated the cells with 1 . Combined treatment with siMBNL1 (which reduced the level of MBNL1 mRNA by ~70% relative to untreated controls) and compound 1 allowed us to test whether reducing the pool of available MBNL1 exerts any effects on the splicing dysregulation induced by 1 and to assess whether 1 induces DM1-like splicing shift via MBNL1-dependent mechanism. Importantly, compound 1 -induced dysregulation of pre‐mRNA alternative splicing of MBNL1-regulated exons ( MBNL1 , MBNL2 , NCOR2 and NFIX ) was significantly exacerbated by MBNL1 knockdown, strongly suggesting that the effects of 1 are indeed MBNL1-dependent ( Fig. 5 ). For all analysed MBNL1-regulated exons, splicing changes induced by highest concentration of 1 (that is, 500 μM) combined with an siRNA against MBNL1 were much more pronounced than those induced by 1 alone ( Figs 4 and 5 ). We hypothesize that knocking-down MBNL1 with siRNA makes it possible to ‘saturate’ the remaining pool of MBNL1 with compound 1 , and thus augments the effect of 1 on the alternative splicing dysregulation of MBNL1-regulated exons. 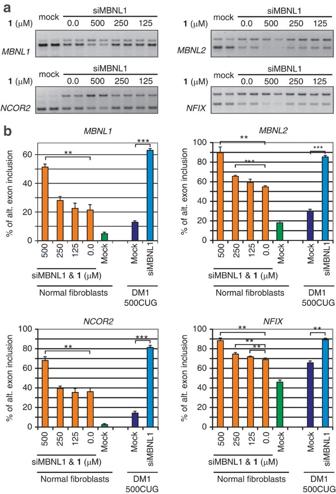Figure 5:MBNL1knockdown exacerbates DM1-like splicing shift induced by compound1in normal human fibroblasts. (a) Representative RT–PCR assays showing splicing changes in MBNL1-dependent exons of four genes in normal fibroblasts treated with siRNA against MBNL1 (siMBNL1) and increasing amounts of1(n=2). Mock controls are lipofectamine-treated samples. (b) Quantification of alternative splicing shift towards the DM1-like phenotype (% of alternative exon inclusion) in four MBNL1-regulated exons (MBNL1, MBNL2, NCOR2andNFIX) upon combined treatment of normal human fibroblasts with an siRNA against MBNL1 and increasing concentrations of1(orange bars;n=2). For comparison, splicing shifts in siMBNL1-treated DM1 affected 500CUG fibroblasts are shown (blue bars;n=2). Mock controls represent splicing changes in lipofectamine-treated cells (green bars—normal fibroblasts; violet bars—500CUG fibroblast;n=2). ‘*’ indicatesP≤0.05; ‘**’ indicatesP≤0.01; and ‘***’ indicatesP≤0.001 as determined by a two-tailed Student’st-test. Figure 5: MBNL1 knockdown exacerbates DM1-like splicing shift induced by compound 1 in normal human fibroblasts. ( a ) Representative RT–PCR assays showing splicing changes in MBNL1-dependent exons of four genes in normal fibroblasts treated with siRNA against MBNL1 (siMBNL1) and increasing amounts of 1 ( n =2). Mock controls are lipofectamine-treated samples. ( b ) Quantification of alternative splicing shift towards the DM1-like phenotype (% of alternative exon inclusion) in four MBNL1-regulated exons ( MBNL1, MBNL2, NCOR2 and NFIX ) upon combined treatment of normal human fibroblasts with an siRNA against MBNL1 and increasing concentrations of 1 (orange bars; n =2). For comparison, splicing shifts in siMBNL1-treated DM1 affected 500CUG fibroblasts are shown (blue bars; n =2). Mock controls represent splicing changes in lipofectamine-treated cells (green bars—normal fibroblasts; violet bars—500CUG fibroblast; n =2). ‘*’ indicates P ≤0.05; ‘**’ indicates P ≤0.01; and ‘***’ indicates P ≤0.001 as determined by a two-tailed Student’s t -test. Full size image In agreement with our hypothesis, the combined effect of siMBNL1 and 500 μM 1 in normal fibroblast resulted in a roughly similar level of splicing shifts as those induced by MBNL1 knockdown in DM1‐affected fibroblasts expressing 500 r(CUG) repeats (500CUG fibroblasts) ( Fig. 5 ). Likewise, 500CUG fibroblasts showed augmented pre‐mRNA alternative splicing dysregulation of MBNL1 , MBNL2 , NCOR2 and NFIX exons when treated with high concentration of 1 alone (that is, 400 μM but not 200 μM) ( Supplementary Figs S4–S7 ). The extent of MBNL1 and MBNL2 splicing dysregulation in these cells was similar to DM1‐affected cells that express 1,000 or 2,000 r(CUG) repeats, and reached the level observed in normal fibroblasts treated with siMBNL1 ( Fig. 4b and Supplementary Fig. S3 ). Taken together, these data strongly support our hypothesis that the DM1-like splicing shift exerted by 1 is mediated via MBNL1-dependent mechanism. To investigate the specificity of 1 towards MBNL1 activity, we analysed the effects of the compound on the alternative splicing of seven exons regulated independently of MBNL1, rather controlled by the splicing regulators MBNL2, polypyrimidine tract-binding protein 1 (PTBP1) or neuro-oncological ventral antigen 1 (NOVA1). Importantly, 1 did not affect the alternative splicing of previously established MBNL2-dependent exons of casein kinase 1 delta ( CSNK1D ), spectrin alpha chain, non-erythrocytic 1 ( SPTAN1 ) and coactivator-associated arginine methyltransferase 1 ( CARM1 ) even though MBNL1 and MBNL2 show high similarity of amino-acid sequence ( Fig. 4c and Supplementary Fig. S8 ) (refs 29 , 30 ). Furthermore, the splicing of NOVA1-dependent exons of mitogen‐activated protein kinase kinase kinase kinase 4 ( MAP4K4 ) and amyloid beta (A4) precursor‐like protein 2 ( APLP2 ) as well as PTBP1-regulated exons of polypyrimidine tract-binding protein 2 ( PTBP2 ) and fibroblast growth factor receptor 1 ( FGFR1 ) were also unaffected in normal human fibroblasts treated with 1 ( Fig. 4c and Supplementary Fig. S8 ). To confirm that the exons under investigation are regulated independently of MBNL1, we analysed their alternative splicing upon siRNA-mediated MBNL1 knockdown in normal and DM1 affected human fibroblasts. Indeed, none of these exons showed significantly altered splicing pattern upon siRNA knockdown of MBNL1 ( Supplementary Fig. S3 ). Intriguingly, however, DM1 affected fibroblasts expressing 2,000 r(CUG) repeats displayed marked splicing shift in PTBP2 when compared with compound 1 -treated normal human fibroblasts, even though siRNA knockdown experiments have shown that this particular splicing event is apparently MBNL1-independent ( Fig. 4c and Supplementary Figs S3 and S8 ). Our interpretation of these results is that DM1 affected cells, in addition to MBNL1 sensitivity, might have additional inherent differences in their ability to regulate MBNL1-independent splicing events, for example via CUGBP1 or other splicing regulators. This hypothesis is bolstered by a recent report by Jog et al . [31] in which they show that number and severity of alternative pre-mRNA splicing defects is reflective of the amount of free MBNL1. That is, modest changes in repeat number or the extent of r(CUG) exp hairpin structure formation (and thus the amount of active MBNL1) causes phenotypic variations [31] . Taken together, our data strongly suggest that 1 specifically affects the function of MBNL1 protein in vivo . Compound 2 improves splicing defects In contrast, compound 2 improves DM1-associated pre-mRNA splicing defects in HeLa cells transfected with the DM1 mini-gene ( Fig. 6 ). Addition of as little as 125 μM of 2 to cells that express r(CUG) exp restores IR pre-mRNA splicing back to levels those observed in the absence of r(CUG) exp . Similarly, improvement in cTNT alternative splicing is also observed. When cells are treated with 300 μM of 2 , pre-mRNA splicing levels are statistically indistinguishable from those observed in the absence of r(CUG) exp and thus are statistically different from cells that express r(CUG) exp . 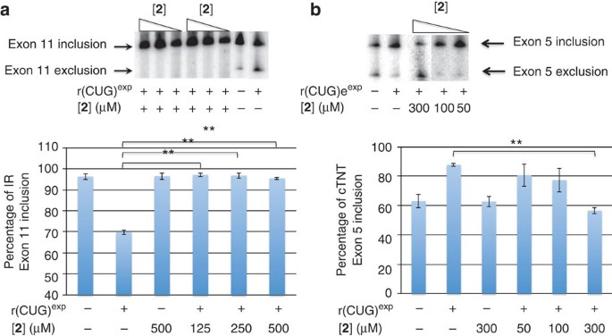Figure 6: Compound2improves DM1-like splicing defects induced in HeLa cells. (a) Compound2improves dysregulation of IR alternative splicing in a DM1 model cellular system. (a, top) Representative gel image of IR alternative splicing in the presence of varying concentrations of2. (a, bottom) Quantification of exon inclusion for IR alternative splicing in the presence or absence of r(CUG)expand2(n≥3). Error bars are the s.d. values in the measurements. (b) Compound2improves dysregulation of cTNT alternative splicing in a DM1 model cellular system. (b, top) Representative gel image of cTNT alternative splicing in the presence of varying concentrations of2. (b, bottom) Quantification of exon inclusion for cTNT alternative splicing in the presence or absence of r(CUG)expand2(n≥3). Error bars are the s.d. values in the measurements. The percentage of each isoform was determined by RT–PCR using a radioactively labelled forward PCR primer. ‘**’ indicatesP≤0.01 as determined by a two-tailed Student’st-test. Figure 6: Compound 2 improves DM1-like splicing defects induced in HeLa cells. ( a ) Compound 2 improves dysregulation of IR alternative splicing in a DM1 model cellular system. ( a , top) Representative gel image of IR alternative splicing in the presence of varying concentrations of 2 . ( a , bottom) Quantification of exon inclusion for IR alternative splicing in the presence or absence of r(CUG) exp and 2 ( n ≥3). Error bars are the s.d. values in the measurements. ( b ) Compound 2 improves dysregulation of cTNT alternative splicing in a DM1 model cellular system. ( b , top) Representative gel image of cTNT alternative splicing in the presence of varying concentrations of 2 . ( b , bottom) Quantification of exon inclusion for cTNT alternative splicing in the presence or absence of r(CUG) exp and 2 ( n ≥3). Error bars are the s.d. values in the measurements. The percentage of each isoform was determined by RT–PCR using a radioactively labelled forward PCR primer. ‘**’ indicates P ≤0.01 as determined by a two-tailed Student’s t -test. Full size image Fluorescence in situ hybridization was employed to determine if 2 decreases the number or intensity of nuclear foci. Although foci are still present, they are much more dispersed when cells are treated with 2 , and it appears that there is less MBNL1 within the foci as determined by immunostaining (MB1a antibody ( Supplementary Fig. S9 and Supplementary Note 1) (ref. 32 ). To test the specificity of splicing modulation by compound 2 , we examined its effect on exons not regulated by MBNL1. HeLa cells were co-transfected with a DM1 mini-gene and splicing reporter constructs for PLEKHH2 , SMN2 and Bcl-x , the alternative splicing of which have been shown previously not to be regulated by MBNL1 (refs 5 , 26 , 27 , 28 ). Treatment with 500 μM 2 had no effect on the alternative splicing of PLEKHH2 , SMN2 or Bcl-x mini-genes ( Supplementary Fig. S2 a–c), regardless of whether cells expressed r(CUG) exp . The alternative splicing of endogenous mRNAs not regulated by MBNL1, CAMKK2 (calcium/calmodulin-dependent protein kinase kinase 2) and TTC8 (tetratricopeptide repeat domain 8) (ref. 26 ), were also not affected ( Supplementary Fig. S2 d,e). Thus, the effect of compound 2 appears to be specific to its ability to bind r(CUG) exp and displace MBNL1. Next, we determined if 2 also improves defects associated with MBNL2 sequestration by r(CUG) exp as they contribute to toxicity in the central nervous systems/brains of DM1 patients [29] . For this purpose, the HEK cell line was used as it expresses MBNL proteins at very low levels [33] . HEK cells were co-transfected with the DM1 and cTNT mini-genes and increasing amounts of a plasmid encoding MBNL1 or MBNL2. As expected, increased expression levels of MBNLs suppress cTNT exon 5 inclusion [10] , [23] , confirming that cTNT alternative splicing is regulated by both proteins in our model system ( Supplementary Fig. S10 ). Dysregulation of cTNT alternative splicing is improved when HEK cells that express r(CUG) exp and MBNL1 or MBNL2 are treated with 300 μM of 2 , although the effect is somewhat less for splicing regulated by MBNL2 ( Supplementary Fig. S11 ). (Dysregulation of splicing is not improved when cells are treated with 75 μM or 150 μM of 2 .) Taken together, 2 inhibits r(CUG) exp –MBNL1 and r(CUG) exp –MBNL2 complexes. Molecular modelling and docking studies A set of docking studies support our experimental evidence that 1 binds to MBNL1 and 2 binds to r(CUG) repeats. 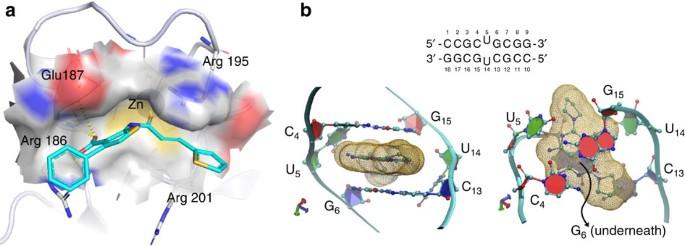Figure 7: Docking studies support the binding of1to MBNL1 and2to r(CUG) repeats. (a) Extensive interactions are observed between MBNL1 and1at the RNA-binding pocket. The ethenyl group and the phenyl and thiofuran rings of1are stabilized by extensive cation–π interactions with arginine residues. The cation–π interaction between1and Arg195 is reminiscent of the MBNL1–RNA interaction34. The ligand binding pocket is shown as a transparent surface. Hydrogen bonds are shown as yellow dash lines. (b) Lowest free energy conformation of the2–r(CUG) complex (binding mode p inSupplementary Table S5andSupplementary Fig. S13). (b, top) RNA sequence used in MD simulations. Side (b, bottom left) and top (b, bottom right) views of the2–r(CUG) complex. The yellow wireframe represents the molecular surface of compound2. The RNA backbone is represented in light blue. For simplicity, hydrogen atoms are not shown. Note that in this binding mode, the interactions in the UU pair (green) are fully lost, and compound2stacks between the flanking GC base pairs (represented in red and blue). Figure 7a shows the results of the molecular modelling of 1 and MBNL1. The model of the complex shows extensive interactions between MBNL1 and 1 that occurs in the RNA-binding pocket. The ethenyl group and the phenyl and thiofuran rings of 1 are stabilized by extensive cation–π interactions with Arg186, Arg195 and Arg201. The cation–π interaction between 1 and Arg195 is reminiscent of the interaction between MBNL1 and RNA [34] . In addition, compound 1 ’s carboxyl group forms a bifurcated hydrogen bond with backbone amino groups of Arg186 and Glu187, as well as a hydrogen bond with side chain of Arg186. Noticeably, the carbonyl oxygen of 1 is within the coordination distance of a bound Zn ion. This suggests that the oxygen provides the fifth coordination site, completing the trigonal bipyramidal geometry of the Zn ion. Figure 7: Docking studies support the binding of 1 to MBNL1 and 2 to r(CUG) repeats. ( a ) Extensive interactions are observed between MBNL1 and 1 at the RNA-binding pocket. The ethenyl group and the phenyl and thiofuran rings of 1 are stabilized by extensive cation–π interactions with arginine residues. The cation–π interaction between 1 and Arg195 is reminiscent of the MBNL1–RNA interaction [34] . The ligand binding pocket is shown as a transparent surface. Hydrogen bonds are shown as yellow dash lines. ( b ) Lowest free energy conformation of the 2 –r(CUG) complex (binding mode p in Supplementary Table S5 and Supplementary Fig. S13 ). ( b , top) RNA sequence used in MD simulations. Side ( b , bottom left) and top ( b , bottom right) views of the 2 –r(CUG) complex. The yellow wireframe represents the molecular surface of compound 2 . The RNA backbone is represented in light blue. For simplicity, hydrogen atoms are not shown. Note that in this binding mode, the interactions in the UU pair (green) are fully lost, and compound 2 stacks between the flanking GC base pairs (represented in red and blue). Full size image We previously reported the structure of r(CCGCUGCGG) 2 , which was determined by NMR spectroscopy [35] . These studies showed that the UU mismatch stacks within the helix, maintaining an overall A-form geometry. The UU mismatch is dynamic, however, and can interconvert between structures that contain 0, 1 or 2 hydrogen bonds [35] . This dynamic nature could provide a means for small molecule binding. Docking studies of 2 and a r(CUG) repeat were completed using the structure of r(CCGCUGCGG) 2 . (Because of the dynamic nature of the RNA, a new method to simulate the binding of 2 to r(CUG) repeats was developed ( Supplementary Methods ). The lowest free energy conformation of the 2 –r(CUG) complex is shown in Fig. 7b . The complex is stabilized by stacking of 2 on the 5′ and 3′ closing GC pairs (shown in red and blue, respectively; Fig. 7b ) and formation of three hydrogen bonds with the uridine bases. Both of 2 ′s amino groups hydrogen bond with one uridine base: one hydrogen bonds with the uridine’s N1 while the other hydrogen bonds with a non-bridging oxygen. Compound 2 ′s nitrile N hydrogen bonds with another U’s H2′. Non-canonical 1 × 1 UU base pairs have weaker hydrogen bonds compared with Watson–Crick base pairs, which makes them more sensitive to the environment such as in the presence of 2 . The pathway for the binding mode shown in Fig. 7b is via the minor groove side as no major groove side binding was seen in the molecular dynamics simulation trajectories ( Supplementary Figs S13 and S14 and Supplementary Note 2). Initial contact between 2 and the UU mismatch occurs at the minor groove side where 2 ′s amino groups interact with the free carboxyl group of the uridine bases. While compound 2 tries to stack within the helix, the weak hydrogen bonds of the UU mismatch break, resulting in one of the uridines unstacking from the helix. Later, the second uridine unstacks from the helix and yields the final binding mode where 2 is fully stacked between the flanking GC base pairs ( Fig. 7b ). The simulation indicates that the complex is dynamic ( Supplementary Figs S13 and S14 ) and that stacking is the predominant interaction driving complex formation. Only very few compounds have been previously reported to target the protein in an RNA–protein complex. A notable example includes the development of T5626448, a small molecule that inhibits the formation of the toll-like receptor 3–dsRNA complex [36] . This interaction activates toll-like receptor 3 and causes induction of pro-inflammatory cytokines. Interestingly, T5626448 shares several similar chemotypes with 1 ; both have carboxylate groups and thiophene-like side chains. Collectively, these data suggest that these chemotypes may be biased for targeting Zn-finger-containing proteins that form RNA–protein complexes. Previous studies have shown that a variety of small molecules bind the expanded triplet repeat in the r(CUG) exp –MBNL1 complex and improve pre-mRNA splicing and other defects in cellular models of DM1. For example, both pentamidine and a bis -benzimidazole improve pre-mRNA splicing defects in DM1 cellular model systems and a transgenic mouse model [26] , [37] . These compounds have modest potencies with pentamidine requiring dosage of 25 μM and the bis -benzimidazole requiring dosage of 100 μM in cellular models. Modularly assembled small molecules that target the repeating 5′C U G/3′G U C motifs in r(CUG) exp require lower concentrations (as low as 5 μM) to improve splicing and translational defects in cellular models [17] , [38] . Thus, even though 2 is a modestly potent modulator of r(CUG) exp toxicity, its bioactivity could be enhanced via modular assembly. It is likely that sites in 2 can be identified to enable such an approach, perhaps via reduction of the cyano group to an amine handle. Compound 2 is more selective than previously reported small molecules that bind to expanded repeats. It binds with ~11-fold selectivity for an RNA that displays 12 5′C U G/3′G U C motifs when compared with an RNA that displays 12 5′C A G/3′G A C and >200-fold selectivity over a fully paired RNA ( Table 2 ). A bis -benzimidazole that also improves DM1-associated defects shows at best threefold selectivity for RNAs with a single 5′C U G/3′G U C (ref. 37 ). A 4′,6-diamidino-2-phenylindole derivative binds to r(CAG) exp and improves associated pre-mRNA splicing defects [39] . This compound has modest specificity for the 5′C A G/3′G A C motif displayed by r(CAG) exp , ranging from ~2-5 fold selectivity over RNAs that display other 1 × 1 nucleotide mismatches and >10-fold selectivity over fully paired RNAs [39] . Compounds 1 and 2 have utility as probes and tools. The ability to reverse or induce a disease-like state chemically can enable studies to determine the repertoire of pre-mRNAs whose splicing function is dysregulated in DM1 or other diseases by using RNA-seq. Studies could also be completed in animal models of DM1, such as in Drosophila , to determine if 1 can induce DM1-like pre-mRNA splicing defects. The compound can then be withdrawn to measure recovery back to wild type. Lastly, these compounds could have a use in the development of artificial gene circuits. Traditionally, such circuits have been controlled through aptamer-small molecule interactions in which the aptamer has been selected or excised from a riboswitch [40] , [41] , [42] , [43] . Compounds Compounds 1 and 4 were procured from Enamine (catalogue numbers T0306-5218 and T0504-3845, respectively). Compound 2 was purchased from eMolecules (Specs) (catalogue number AN-584/43420506), and compound 3 was purchased from Vitas-M Laboratory, Ltd (catalogue number STK676326). All compounds were >95% pure. Competition dialysis Competition dialysis was completed as described previously [18] . Briefly, 5′-biotinylated r(CUG) 12 , MBNL1 protein and BSA were diluted separately to a final concentration of 2.5 μM in 1 × phosphate buffer EDTA saline (1 × PBES, 8 mM Na 2 HPO 4 (pH=7.0), 185 mM NaCl, 1 mM EDTA). The RNA was folded by heating at 60 o C for 5 min and slow cooling to room temperature. Compound 1 was then added at a final concentration of 2.5 μM to the folded RNA, MBNL1 or BSA solution. A 150 μl aliquot of each solution was added to a dialysis unit (Pierce Slide-A-Lyzer MINI dialyzer unit (7000, kDa MWCO; Pierce Biotechnology, Inc.). Dialysis units were placed in 200 ml of dialysate, which consisted of 2.5 μM of 1 in 1 × PBES. The samples were allowed to equilibrate with dialysate by stirring at 70 r.p.m. for 48 h at room temperature (20–22 ° C). At the end of the equilibration period, sodium dodecyl sulphate (SDS) was added to the sample solution to the final concentration of 1% (v/v). Addition of SDS was necessary to ensure complete dissociation of 1 from the RNA or protein, as binding can affect its spectroscopic properties. The total concentration of 1 ( C t ) within the dialysis unit was determined spectrophotometrically using an appropriate absorbance wavelength and extinction coefficient. A dilution factor was applied to account for the addition of SDS. The free concentration of 1 ( C f ) was determined from an aliquot of the dialysate solution, which did not vary appreciable from the initial 2.5 μM. The bound ligand concentration ( C b ) was then determined using (1) where C b, C t and C f are concentration of 1 in bound, total and free states, respectively. The dissociation constant was determined using (2) (ref. 18 ) [44] : where K app is the apparent association constant (equivalent to 1/ K d ) and [MBNL1] is the concentration of MBNL1. Fluorescence binding assays Dissociation constants of 2 to various 1 × 1 nucleotide internal loops were measured by an in-solution, fluorescence-based assay. RNA was folded in 1 × PBES at 60 ° C for 5 min and allowed to slowly cool to room temperature. 2 was then added to a final concentration of 1,250 nM. This solution was then serially diluted (2 × ) into 1 × PBES solution containing 1,250 nM of 2 . The solutions were incubated at room temperature for 10 min and then transferred to a 96-well plate. Anisotropy signal was recorded using a Spectra Max M5 plate reader (excitation 300 nm; emission: 470 nm; cutoff: 420 nm). The change in anisotropy signal as a function of RNA concentration was fitted to a standard ligand binding for one site saturation for r(CAG) 12 , 1 × 1 UU and AU RNAs (3): where Δ r is the change in anisotropy signal, B max represents the maximum number of binding sites, [ RNA ] is the RNA concentration and K d is the dissociation constant. The dissociation constant for binding to r(CUG) 12 was determined via a Hill plot. RNA-MBNL1 displacement assays The RNA-MBNL1 binding studies were completed as previously described [37] , [39] . Briefly, 5′-biotinylated r(CUG) 12 (folded by heating at 60 ° C for 5 min then slowly cooling to room temperature) or MBNL1-His 6 was incubated with compound for 30 min at room temperature. Next, r(CUG) 12 was added to MBNL1-containing samples or vice versa, and the samples were incubated for 15 min at room temperature. Streptavidin-XL665 (binds to the biotinylated RNA oligonucleotide) and Tb-Anti-His 6 (binds to MBNL1) were then added. After 1 h, TR-FRET was measured using a Molecular Devices SpectraMax M5 plate reader. IC 50 ’s were determined by fitting the corresponding curve to SigmaPlot’s four parameter logistic curve fit. Assessment of DM1-associated translational defects The model systems used to study the DM1-associated translational defect have been previously described [17] . Briefly, a C2C12 cell line that stably expresses the firefly luciferase gene containing a (CTG) 800 expansion in the 3′-UTR was employed. r(CUG) 800 causes nuclear retention of the luciferase mRNA and thus decreased expression of luciferase. Compounds that disrupt the r(CUG) 800 –MBNL1 interaction, therefore, have the potential to allow for nucleocytoplasmic export, which is correlated to the luciferase activity in cell extracts. Cells were treated with compound for 16 h and then lysed. Luciferase activity was measured using a Luciferase Assay Kit (Promega) as previously described [17] . Assessment of pre-mRNA splicing defects in cellular models DM1-associated pre-mRNA splicing defects using a HeLa model system were completed as previously described [17] , [26] , [37] using a DM1 mini-gene that expresses 960 interrupted r(CUG) repeats [10] . Briefly, HeLa cells were co-transfected with the mini-gene of interest and a plasmid that expresses r(CUG) exp or an empty vector. Varying concentrations of compound were added in growth medium post transfection, and total RNA was harvested 16–20 h later. The percentage of each splicing isoform was determined by RT–PCR. Statistical significance was determined using a two-tailed Student's t -test. HEK 293T cells were grown as monolayers in 96-well plates to ~95% confluency in growth medium (1 × DMEM, 10% FBS, and 1 × GlutaMax (Invitrogen)). In order to show that the cTNT mini-gene was responsive to MBNL1 and MBNL2 in the HEK model system, cells were co-transfected with plasmids expressing the DM1 mini-gene (100 ng), the cTNT mini-gene (100 ng) and MBNL1 or MBNL2 (varying amounts; 0–60 ng) using Lipofectamine 2000 reagent as per the manufacturer’s protocol. The effects of compound 2 on MBNL1- and MBNL2-dependent alternative splicing were then determined using 100 ng DM1 mini-gene plasmid, 100 ng cTNT mini-gene plasmid and 5 ng of MBNL plasmid. Approximately 5 h post transfection, the transfection cocktail was replaced with growth medium containing various concentrations of 2 (0, 75, 150 and 300 μM). After 16–24 h, the cells were lysed, and total RNA was collected using a GelElute Mammalian Total RNA Miniprep Kit (Sigma-Aldrich). RT–PCR analysis was completed as previously described [17] , [26] , [37] . DM1 patient-derived cell lines and compound 1 treatment The following cell lines were obtained from the Coriell Cell repositories: GM07492—fibroblasts from unaffected individual (normal fibroblasts); GM03987, GM04033 and GM03989—fibroblasts from DM1 probands expressing mutant DMPK transcript containing ~500, ~1,000 and ~2,000 CUG repeat tracts, respectively (referred to as 500CUG, 1000CUG and 2000CUG, respectively). Cells were grown in a high-glucose EMEM (Lonza) supplemented with 10% fetal bovine serum, 1 × antibiotic-antimycotic (Gibco) and 1 × non-essential amino acids solution (Sigma), in a humidified incubator containing 5% CO 2 , at 37 °C. Appropriate amounts of compound 1 were mixed with medium and added directly to 70–80% confluent cells. All splicing changes were analysed 48 h post treatment. siRNA knockdown of MBNL1 siRNA oligos targeting human MBNL1 were obtained from Future Synthesis, and the sequences were as follows: MBNL1_AS 5′[P]-UCUCUACAUACUUCCAGUGdTdT, MBNL1_S 5′[P]-CACUGGAAGUAUGUAGAGAdTdT [31] . At 80% confluence, fibroblasts were transfected with 25 nM annealed siRNA directed against MBNL1 transcript (referred to as siMBNL1) using Lipofectamine 2000 (Invitrogen). All splicing changes were analysed 48 h post siMBNL1 treatment. For combined siMBNL1 and compound 1 treatment, normal human fibroblasts were successively treated with 25 nM siMBNL1 and 125, 250 or 500 μM compound 1 . Cells were first transfected with 25 nM siMBNL1 at 70–80% confluence. Then, appropriate amounts of compound 1 were added 24 h post siMBNL1 treatment. The following controls were used for combined siMBNL1 and 1 treatment: lipofectamine-treated cells (mock), siMBNL1 only, and compound 1 only treated cells. All splicing changes were analysed 48 h post compound 1 treatment (72 h post siMBNL1 treatment). RNA isolation and RT–PCR RNA was isolated 48 h post 1 treatment or siRNA treatment using TRI reagent (Sigma-Aldrich) per the manufacturer’s recommended protocol. cDNA was synthesized using SuperscriptTM III Reverse Transcriptase kit (Invitrogen) according to the manufacturer’s protocol, and diluted with 50 μl water before PCR. Standard RT–PCR reactions were performed using 2 μl diluted cDNA and GoTaq Flexi DNA Polymerase kit (Promega). PCR primer sequences are listed in Supplementary Table S1 . PCR products were separated on a 2% agarose gel stained with 0.5 μg ml −1 ethidium bromide, photographed using G-Box (SynGene) and quantified with the use of GeneTools Software (SynGene). Quantified splicing changes were plotted on a bar graph as a percentage of the respective exon spliced in (% of alternative exon inclusion), which in the case of MBNL1-dependent exons represents splicing isoforms characteristic of DM1. Experimental set-up and statistical analyses The effect of 1 on normal and DM1 (CUG500) human fibroblasts was analysed in duplicate biological repeats ( n =2 for each given concentration of 1 ). As controls, we used n =5 each for untreated and DMSO-treated normal human fibroblasts, and n =2 for the untreated CUG500 fibroblasts. For additional DM1 controls, we used n =4 each of the untreated CUG1000 and CUG2000 human fibroblasts. The effects of siMBNL1 knockdown as well as combined siMBNL1 and compound 1 treatment were assessed in duplicate biological repeats. All RT–PCR reactions were performed and analysed at least twice to verify results. The fractions of alternatively spliced isoforms (exon inclusions representing the DM1-like splicing isoform) were calculated by dividing the intensity of a PCR product band corresponding to the splicing variant representing exon inclusion (upper band) by the total intensity of both splicing isoforms (upper and lower band). Error bars represent s.d. (±s.d.) obtained from a single experiment with at least two independent biological repeats. Statistical significance was determined by a two-tailed Student’s t -test using Microsoft Excel (* for P ≤0.05, ** for P ≤0.01 and *** for P ≤0.001). Docking of 1 and MBNL1 Compound 1 was prepared for docking simulations using LigPrep v2.5 (Schrodinger, LLC) [44] , affording a single ligand pose. PDB entry 3D2S (MBNL1) was prepared for molecular modelling by using Maestro’s protein preparation wizard (v9.3; Schrodinger, LLC). Bound RNA and water molecules were removed, the bond order was assigned, and hydrogen atoms were added. The rotamer states of Asn and Gln residues, and the charge states of His residues were also optimized. The docking grid was generated around the Zn coordinate with a box size of 15 × 15 × 15 Å 3 . No constraints were used for grid generation. Compound 1 was then docked into MBNL1 ref. 34 using Glide SP v5.6 (Schrodinger, LLC). Energy minimization was completed using Prime v3.1 under the Maestro interface (Schrodinger, LLC). Figure 7a was generated using PyMol (Schrodinger, LLC). Docking of 2 and r(CUG) repeats Please see the Supplementary Methods and Supplementary Tables S2-S5. for details related to molecular modelling of 2 and r(CUG) repeats. How to cite this article: Childs-Disney, J. L. et al . Induction and reversal of myotonic dystrophy type 1 pre-mRNA splicing defects by small molecules. Nat. Commun. 4:2044 doi: 10.1038/ncomms3044 (2013).